Constitutive phospholipid scramblase activity of a G protein-coupled receptor Opsin, the rhodopsin apoprotein, was recently shown to be an ATP-independent flippase (or scramblase) that equilibrates phospholipids across photoreceptor disc membranes in mammalian retina, a process required for disc homoeostasis. Here we show that scrambling is a constitutive activity of rhodopsin, distinct from its light-sensing function. Upon reconstitution into vesicles, discrete conformational states of the protein (rhodopsin, a metarhodopsin II-mimic, and two forms of opsin) facilitated rapid (>10,000 phospholipids per protein per second) scrambling of phospholipid probes. Our results indicate that the large conformational changes involved in converting rhodopsin to metarhodopsin II are not required for scrambling, and that the lipid translocation pathway either lies near the protein surface or involves membrane packing defects in the vicinity of the protein. In addition, we demonstrate that β 2 -adrenergic and adenosine A 2A receptors scramble lipids, suggesting that rhodopsin-like G protein-coupled receptors may play an unexpected moonlighting role in re-modelling cell membranes. Polar lipids must flip rapidly across biological membranes to sustain cellular life. For example, phospholipids such as phosphatidylcholine (PC) are synthesized on the cytoplasmic face of the endoplasmic reticulum (ER) and must be apportioned between the luminal and cytoplasmic leaflets for uniform expansion of the ER during cell growth [1] , [2] , [3] , [4] . Transbilayer movement of phospholipids is also needed to generate, maintain and dissipate the physiologically important transbilayer lipid asymmetry of the plasma membrane [5] , [6] , [7] . As flipping is energetically costly [8] , [9] , specialized transporters are needed to increase its intrinsically low rate to a physiologically appropriate level [10] . Some of these transporters are ATPases that couple lipid translocation to ATP hydrolysis [5] , [6] , [11] , whereas others function without any discernible metabolic energy input. The molecular identity of these latter ‘ATP-independent flippases’, also termed ‘scramblases’, has eluded researchers for decades and only recently have members of this class of proteins been identified and their activity verified by reconstitution into phospholipid vesicles [12] , [13] , [14] . Rod photoreceptor discs in mammalian retina are host to a variety of lipid translocation events that are necessary for maintaining the functionally important transbilayer lipid asymmetry of the disc membrane, and for preventing the accumulation of toxic retinoid compounds implicated in forms of age-related macular degeneration and genetic blinding diseases such as Stargardt’s and Best disease [11] , [13] , [15] , [16] , [17] , [18] , [19] , [20] . Thus, discs contain ABCA4, an ABC transporter implicated in the transbilayer transport of a retinoid-phosphatidylethanolamine (PE) adduct [17] , [21] , as well as Atp8a2, a P 4 -ATPase that moves phosphatidylserine from the disc’s interior to its cytoplasmic face [15] . Both of these proteins couple lipid movement to ATP hydrolysis. In addition, as originally reported by Wu and Hubbell [22] , and Hofmann and co-workers [23] , [24] , phospholipids flip-flop rapidly and bidirectionally across bovine photoreceptor discs in an ATP-independent manner. The rates of inward and outward translocation were found to be similar, and fast, such that phospholipid probes could equilibrate across the disc bilayer within minutes. We recently reported that ATP-independent flip-flop of phospholipids in discs is due to opsin [13] , the apoprotein of the G protein-coupled receptor (GPCR) rhodopsin that is responsible for light sensation [13] , [25] , [26] : upon reconstitution into large unilamellar vesicles, opsin facilitates rapid, ATP-independent flip-flop of common phospholipids. In our original report we described opsin as an ATP-independent phospholipid flippase; we now refer to it by the equivalent term ‘phospholipid scramblase’. Opsin is the first phospholipid scramblase to be identified and biochemically verified via reconstitution of the purified protein. Very little is known about how such scramblases work. To elucidate opsin’s lipid transport mechanism we considered two questions. Does the presence of retinal regulate opsin-mediated lipid translocation? Are the structurally distinct forms of rhodopsin that are generated by its photoactivation capable of translocating lipids? The first question tests a proposed model of lipid scrambling in which the headgroup of a transiting phospholipid utilizes bulk water within opsin’s transmembrane (TM) heptahelical bundle to provide a low energy path across the membrane, while the lipid’s acyl chains emerge from between TM helices to remain in the membrane interior [13] . Several lines of evidence indicate the presence of substantial amounts of water inside the protein [27] , [28] , [29] , [30] , [31] . The presence of retinal would affect the amount of internal water and would be predicted to block transport in this model. The second question probes the overall structural requirements for lipid scrambling and investigates whether scrambling activity is linked to phototransduction. To address these questions we generated three structurally distinct forms of bovine rhodopsin and assayed their ability to scramble phospholipids. We prepared inactive rhodopsin (RhoWT), a constitutively active metarhodopsin II-mimic containing the M257Y mutation (Rho*; ref. 32 ), and the inactive apoprotein opsin (Ops; Fig. 1 ; structural transitions between inactive and active receptor states are reviewed in the study by Ernst et al. [25] ). Rhodopsin has a compact TM heptahelical bundle with its inverse agonist 11- cis -retinal linked to TM helix 7, whereas metarhodopsin II contains the full agonist all- trans -retinal and has a splayed structure in which TM helices 5, 6 and 7 are spread out laterally on the side of the protein that faces the cytoplasm. We also prepared an opsin construct that has enhanced basal activity (Ops*, Fig. 1 ) owing to the M257Y mutation that allows for greater helix dynamics and shifts the equilibrium between inactive and active conformations towards the active state [33] , [34] , [35] . Our results indicate that all three forms of the protein are active in scrambling phospholipids when reconstituted into large unilamellar vesicles. In addition, Ops* that samples both inactive and active conformations was competent to translocate lipids to the same extent as the structurally more discrete forms. We conclude that rhodopsin’s ability to scramble lipids is not linked to its established function as a light-sensing receptor and that the large conformational changes involved in converting rhodopsin to metarhodopsin II (ref. 36 ) are not directly related to the scrambling mechanism. Thus, rhodopsin is a constitutively active phospholipid scramblase. Furthermore, the ability of retinal-containing constructs (RhoWT and Rho*) to scramble lipids suggests that the lipid translocation path does not involve the water-containing central core of the protein. 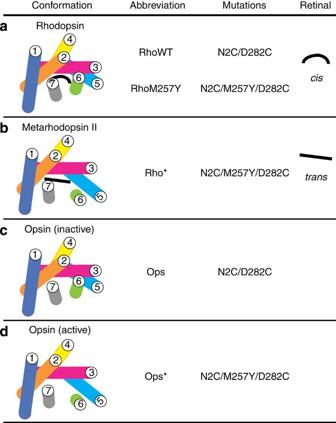Figure 1: Conformational states of rhodopsin analyzed in this study. The cartoon representations show the cytoplasmic face of the proteins: (a) inverse agonist-bound rhodopsin, (b) agonist-bound metarhodopsin II, (c) inactive and (d) active forms of the apoprotein opsin. The N2C/D282C double mutation confers thermostability, and the M257Y mutation generates a mimic of metarhodopsin II. Figure 1: Conformational states of rhodopsin analyzed in this study. The cartoon representations show the cytoplasmic face of the proteins: ( a ) inverse agonist-bound rhodopsin, ( b ) agonist-bound metarhodopsin II, ( c ) inactive and ( d ) active forms of the apoprotein opsin. The N2C/D282C double mutation confers thermostability, and the M257Y mutation generates a mimic of metarhodopsin II. Full size image Ops Ops* and Rho* are phospholipid scramblases To determine the phospholipid scramblase activity of different conformational states of bovine rhodopsin, we generated a thermostable N2C/D282C version of the protein [37] ( Fig. 1 ) with a C-terminal 3xFLAG tag to facilitate purification. Ops* and Rho* also contained the constitutively activating M257Y point mutation [32] , [33] . Rho* was generated from purified M257Y rhodopsin by light exposure [32] . Rhodopsins, prepared from Ops- or Ops*-expressing cells that had been incubated with 11- cis -retinal, had the expected light-sensitive absorbance spectra and ability to activate G protein ( Supplementary Fig. 1a,c–e ). As the structure of 11- cis -retinal-containing rhodopsin is virtually indistinguishable from that of 9- cis -retinal-containing isorhodopsin [38] , we used isorhodopsins ( Supplementary Fig. 1b ) for our scramblase analyses unless specified otherwise. We refer to both 9- cis -retinal and 11- cis -retinal regenerated Ops and Ops* as RhoWT and RhoM257Y, respectively. Phospholipid scramblase activity was measured using a previously established assay ( Fig. 2a ) [13] , [39] , [40] in which large unilamellar vesicles containing fluorescent 7-nitro-2,1,3-benzoxadiazol (NBD) acyl-labelled phospholipid reporters symmetrically distributed in both leaflets are treated with dithionite (S 2 O 4 2− ), a negatively charged reducing reagent that cannot cross membranes [41] . Dithionite reduces NBD to 7-amino-2,1,3-benzoxadiazol (ABD) and irreversibly eliminates the fluorescence of NBD-phospholipids situated in the outer leaflet of the vesicles. Thus, on adding dithionite to protein-free NBD-phospholipid-containing vesicles, ~50% of the fluorescence is expected to be lost as outer leaflet NBD lipids are reduced while inner-leaflet lipids are protected. In ‘scramblase-active’ vesicles, all fluorescence should be lost on adding dithionite as flip-flop ensures that inner-leaflet NBD lipids can gain access to the outer leaflet ( Fig. 2a ). 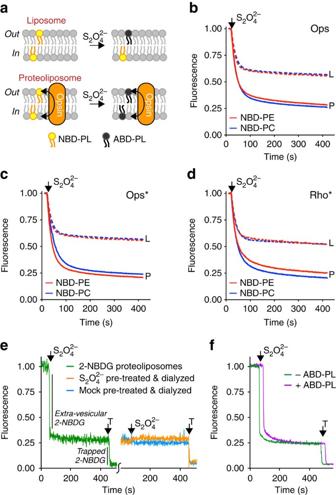Figure 2: Ops Ops* and Rho* flip phospholipids. (a) Schematic representation of the scramblase activity assay. Large unilamellar vesicles are reconstituted with a trace amount of symmetrically distributed NBD-labelled phospholipid (NBD-PL). Dithionite (S2O42−), a membrane-impermeant dianion, reduces NBD-PL to the non-fluorescent ABD-PL. In the absence of a scramblase (top panel) only NBD-PL in the outer leaflet is accessible to S2O42−. In a scramblase (opsin)-containing proteoliposome (bottom panel), NBD-PLs exchange between both leaflets ensuring that even the inner-leaflet pool gains access to dithionite. (b) Scramblase activity of Ops. Representative fluorescence traces corresponding to dithionite treatment of NBD-PE (red) and NBD-PC (blue) containing liposomes (L; dashed lines) and Ops proteoliposomes at a PPR of ~1.5 mg mmol−1(P; solid lines). Dithionite was added att=10 s (arrow) and fluorescence was measured at room temperature with constant stirring for a further 400 s. (c) As inbfor Ops*. (d) As inbfor Rho*. (e) Dithionite cannot reduce intravesicular 2-NBDG. Left, Ops proteoliposomes (PPR~1.5 mg mmol−1) were reconstituted in the presence of 2-NBDG and used directly (‘2-NBDG proteoliposomes’). 2-NBDG fluorescence was recorded over time. Dithionite (S2O42−) was added att=100 s to eliminate fluorescence due to extravesicular 2-NBDG, and Triton X-100 (T) was added at 500 s to disrupt the vesicles. The initial reduction of fluorescence (corresponding to extravesicular 2-NBDG) is less than expected70owing to significant adsorption of 2-NBDG onto Bio-Beads in the course of vesicle reconstitution. Right, Fluorescence traces for ‘2-NBDG proteoliposomes’ that were pre-treated with either dithionite (orange trace) or unbuffered Tris (blue trace) and dialyzed as described in ‘Methods’ before analysis. (f) Dithionite does not cross the membrane of proteoliposomes containing phospholipid probes. Ops proteoliposomes (PPR~1.5 mg mmol−1) were reconstituted with 2-NBDG and with (purple) or without (green) ABD-PC. As observed ine, left, addition of S2O42−att=100 s to both preparations resulted in a comparable TX-sensitive pool of intravesicular 2-NBDG. The traces have been horizontally displaced by 20 s for clarity. Figure 2: Ops Ops* and Rho* flip phospholipids. ( a ) Schematic representation of the scramblase activity assay. Large unilamellar vesicles are reconstituted with a trace amount of symmetrically distributed NBD-labelled phospholipid (NBD-PL). Dithionite (S 2 O 4 2− ), a membrane-impermeant dianion, reduces NBD-PL to the non-fluorescent ABD-PL. In the absence of a scramblase (top panel) only NBD-PL in the outer leaflet is accessible to S 2 O 4 2− . In a scramblase (opsin)-containing proteoliposome (bottom panel), NBD-PLs exchange between both leaflets ensuring that even the inner-leaflet pool gains access to dithionite. ( b ) Scramblase activity of Ops. Representative fluorescence traces corresponding to dithionite treatment of NBD-PE (red) and NBD-PC (blue) containing liposomes (L; dashed lines) and Ops proteoliposomes at a PPR of ~1.5 mg mmol −1 (P; solid lines). Dithionite was added at t =10 s (arrow) and fluorescence was measured at room temperature with constant stirring for a further 400 s. ( c ) As in b for Ops*. ( d ) As in b for Rho*. ( e ) Dithionite cannot reduce intravesicular 2-NBDG. Left, Ops proteoliposomes (PPR~1.5 mg mmol −1 ) were reconstituted in the presence of 2-NBDG and used directly (‘2-NBDG proteoliposomes’). 2-NBDG fluorescence was recorded over time. Dithionite (S 2 O 4 2− ) was added at t =100 s to eliminate fluorescence due to extravesicular 2-NBDG, and Triton X-100 (T) was added at 500 s to disrupt the vesicles. The initial reduction of fluorescence (corresponding to extravesicular 2-NBDG) is less than expected 70 owing to significant adsorption of 2-NBDG onto Bio-Beads in the course of vesicle reconstitution. Right, Fluorescence traces for ‘2-NBDG proteoliposomes’ that were pre-treated with either dithionite (orange trace) or unbuffered Tris (blue trace) and dialyzed as described in ‘Methods’ before analysis. ( f ) Dithionite does not cross the membrane of proteoliposomes containing phospholipid probes. Ops proteoliposomes (PPR~1.5 mg mmol −1 ) were reconstituted with 2-NBDG and with (purple) or without (green) ABD-PC. As observed in e , left, addition of S 2 O 4 2− at t =100 s to both preparations resulted in a comparable TX-sensitive pool of intravesicular 2-NBDG. The traces have been horizontally displaced by 20 s for clarity. Full size image We reconstituted purified proteins (prepared in n -dodecyl-β- D -maltopyranoside (DDM)) together with NBD-PC or NBD-PE into preformed large unilamellar vesicles using a detergent-destabilization procedure. Protein-free vesicles containing the same fluorescent phospholipids were prepared in parallel. On adding dithionite to protein-free vesicles, we observed a rapid 46.7±0.9% (mean±s.e.m., n =8) decrease in fluorescence ( Fig. 2b–d ; dashed traces), consistent with the reduction of outer leaflet NBD-phospholipids; complete reduction was seen after permeabilizing the vesicles with Triton X-100 (TX). The data obtained for NBD-PC and NBD-PE were identical. These results confirm that (i) dithionite does not cross the membrane of protein-free vesicles, and (ii) the NBD-phospholipids are symmetrically reconstituted. We next tested Ops-, Ops*- and Rho*-containing proteoliposomes prepared at a protein-to-phospholipid ratio (PPR) of ~1.5 mg mmol −1 , corresponding to an average of ~12 protein molecules per vesicle. In all three cases, and for both NBD-PE and NBD-PC, ~80% of the fluorescence was lost on adding dithionite, considerably greater than the loss observed with the corresponding protein-free liposomes ( Fig. 2b–d , solid traces). This result suggests that NBD-phospholipids from the inner leaflet of proteoliposomes are flipped to the dithionite-accessible outer leaflet by each of the three protein constructs. We note that despite having many copies of Ops-, Ops*- or Rho* scramblases per vesicle on average, we observed a maximum of 82.6±0.5% ( n =14) loss in fluorescence on adding dithionite ( Fig. 2b–d ) rather than the expected 100%. As previously suggested, this may be because some of the vesicles are refractory to reconstitution, and/or contained within dithionite-resistant aggregates [7] , [12] , [13] , [42] . To rule out the possibility that the greater fluorescence reduction that was observed for proteoliposomes versus liposomes might be due to protein-mediated permeation of dithionite across the membrane rather than scramblase-mediated exposure of inner-leaflet NBD phospholipids at the outer leaflet, we prepared proteoliposomes in the presence of 2-NBD-glucose (2-NBDG). This fluorescent probe is water-soluble and should be trapped within the lumen of the proteoliposomes and thus protected from dithionite. We used the proteoliposomes directly as they were prepared, without separating them from the extravesicular 2-NBDG in the reconstitution buffer. On adding dithionite to the sample ( Fig. 2e , left), the extravesicular 2-NBDG was immediately reduced resulting in a stable fluorescence signal; this fluorescence was due to the intravesicular pool of 2-NBDG, as it was eliminated on adding TX to disrupt the proteoliposomes. To confirm our interpretation of the results, we performed two complementary experiments with proteoliposomes that had been either mock treated or dithionite treated, and then dialyzed prior to analysis ( Fig. 2e , right, blue and orange trace, respectively). In both cases the initial fluorescence intensity was the same as that observed after dithionite treatment of the original proteoliposome preparation. Furthermore, the signal was refractory to dithionite addition but could be eliminated upon addition of TX. To verify that proteoliposomes are not made leaky due to potential interactions between opsin and NBD lipids, we examined whether 2-NBDG was protected in proteoliposomes reconstituted with ABD-PC. This was indeed the case ( Fig. 2f ). The cumulative results demonstrate that neither dithionite nor 2-NBDG are able to cross the proteoliposome membrane during the ~10 min timescale of our assay. Finally, we considered the possibility that the increased fluorescence reduction observed on adding dithionite to proteoliposomes might be due to the asymmetric incorporation of the test proteins that in turn could promote the asymmetric reconstitution of NBD-phospholipids such that ~80% of the NBD-phospholipids are located in the outer leaflet of the vesicles. This was not the case. Collisional quenching of the NBD fluorophore with iodide ions revealed that ~50% of the NBD-phospholipids in proteoliposomes were protected from the quencher, indicating that the lipids were reconstituted symmetrically ( Supplementary Fig. 2a ). Also, protease protection experiments with AspN, an endoprotease that cuts at a single site near the C terminus of opsin, indicated that opsin was symmetrically reconstituted in the vesicles with approximately half the reconstituted protein population resisting AspN proteolysis ( Supplementary Fig. 2b ). These results indicate that the enhanced reduction of NBD-fluorescence observed in proteoliposomes is not a result of asymmetric reconstitution. The cumulative data indicate that all three constructs—Ops, Ops* and Rho*—facilitate transbilayer movement of phospholipids on a timescale of ~100 s. To determine the rate of scrambling more precisely we analyzed the fluorescence reduction time courses ( Fig. 2b–d ) by fitting the traces to a double-exponential function (see ‘Methods’). We found a reproducible fast component ( k fast =0.058±0.0013, s −1 corresponding to a t ½ ~11.9 s ( n =79)) accounting for the majority of the fluorescence change for both protein-free liposomes and proteoliposomes, and a slow component that was not correlated with vesicle protein content over a PPR range of 0.12–1.9 mg mmol −1 (corresponding to 1–16 proteins per vesicle), and that was, on average, more than an order of magnitude slower than the fast component. The origin of the slow component is unknown, but as it is observed in both protein-free liposomes and proteoliposomes it is clearly not related to the flipping process and will not be considered further. The identical fast component seen for both protein-free liposomes and proteoliposomes indicates that the rate of lipid scrambling is similar to, or greater than, that of dithionite-mediated reduction of NBD fluorophores. While this makes it impossible to obtain a precise measure of the lipid translocation rate, we can nevertheless estimate that on a per protein basis, Ops, Ops* and Rho* translocate >10 4 phospholipids per second. Ops Ops* and Rho* reconstitute as multimers To reconstitute proteoliposomes we add proteins to a pre-existing ensemble of phospholipid vesicles, using detergent to destabilize the vesicles to promote protein insertion. The probability ( P (≥1 scramblase)) that any given vesicle in the ensemble acquires at least one functional scramblase as a result of this process, increases monotonically with the amount of protein used for reconstitution. If a single reconstitution event (of protein monomers or multimers) directly confers scramblase activity to the vesicle, then in accordance with Poisson statistics, P (≥1 scramblase) should increase mono-exponentially with PPR (ref. 13 ); thus, P (≥1 scramblase)=1−exp(−PPR/ α ), with α being a fit constant (see ‘Methods’). We can also consider an alternative reconstitution scenario in which two or more reconstitution events are required to confer scramblase activity to a vesicle: here, individual monomers that are reconstituted into a vesicle must subsequently dimerize or multimerize to yield a functional scramblase. In this case, the relationship between P (≥1 scramblase) and PPR would be predicted to be sigmoidal according to the equation P (≥1 scramblase)= P (≥2 reconstitutions into the same vesicle)=1−(1+PPR/ α ) exp(−PPR/ α ). To distinguish between these possibilities, we varied the PPR of our preparations from 0–2 mg mmol −1 and measured the extent of fluorescence reduction on treating the samples with dithionite as in Fig. 2b–d . We did experiments with both NBD-PE and NBD-PC, and transformed the cumulative fluorescence reduction data (see ‘Methods’) to obtain P (≥1 scramblase). Graphs of P (≥1 scramblase) versus PPR for Ops, Ops* and Rho* are shown in Fig. 3a–d . The experimental data in each case are well-described by a mono-exponential function ( Fig. 3a–d , green line) with no indication of sigmoidal behaviour ( Fig. 3b , compare trace 1 (green) and trace 2 (dashed, pink); ‘Methods’), indicating that a single reconstitution event confers scramblase activity to a vesicle. 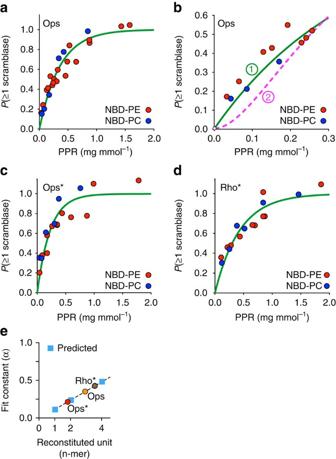Figure 3: Protein-dependence of Ops Ops* and Rho*-mediated phospholipid scrambling. (a) Scramblase activity assays (as inFig. 2b) were done with Ops proteoliposomes prepared with different PPRs using NBD-PE and NBD-PC reporters. The fluorescence reduction data were transformed as described in ‘Methods’13to plot the probability of a vesicle having at least one scramblase,P(≥1 scramblase), versus PPR. The green line through the points is a mono-exponential fit of the cumulative data. (b) Data fromawere fit to either of the two analytical expressions, each with a single fit parameter (α), that describe alternative reconstitution scenarios: a single reconstitution event directly confers scramblase activity to the vesicle ((P(≥1 scramblase)=1−exp(−PPR/α)), or, two or more reconstitution events are required to confer scramblase activity to a vesicle (P(≥1 scramblase)=1−(1+PPR/α) exp(−PPR/α)). The resultant fit constants wereα=0.36 (green line) and 0.16 (pink dashed line) mg mmol−1, respectively, with correspondingχ2-values of 0.15 and 0.35. Thus, the data were better fit by a single exponential consistent with functional scramblase-equipped vesicles being generated via single reconstitution events. (c) as ina, for Ops*. (d) as ina, for Rho*. (e) Graph of the fit constantαfor the equationP(≥1 scramblase)=1−exp(−PPR/α) as a function of the size of the multimer being reconstituted (n-mer). Predicted values for the reconstitution of opsin monomers, dimers, tetramers and octamers are shown as blue squares (the dashed line connecting the squares is intended to guide the eye). Measured fit constants for Ops, Ops* and Rho* (taken from the data ina,c,d) are indicated by filled circles. Figure 3: Protein-dependence of Ops Ops* and Rho*-mediated phospholipid scrambling. ( a ) Scramblase activity assays (as in Fig. 2b ) were done with Ops proteoliposomes prepared with different PPRs using NBD-PE and NBD-PC reporters. The fluorescence reduction data were transformed as described in ‘Methods’ [13] to plot the probability of a vesicle having at least one scramblase, P (≥1 scramblase), versus PPR. The green line through the points is a mono-exponential fit of the cumulative data. ( b ) Data from a were fit to either of the two analytical expressions, each with a single fit parameter ( α ), that describe alternative reconstitution scenarios: a single reconstitution event directly confers scramblase activity to the vesicle (( P (≥1 scramblase)=1−exp(−PPR/ α )), or, two or more reconstitution events are required to confer scramblase activity to a vesicle ( P (≥1 scramblase)=1−(1+PPR/ α ) exp(−PPR/ α )). The resultant fit constants were α =0.36 (green line) and 0.16 (pink dashed line) mg mmol −1 , respectively, with corresponding χ 2 -values of 0.15 and 0.35. Thus, the data were better fit by a single exponential consistent with functional scramblase-equipped vesicles being generated via single reconstitution events. ( c ) as in a , for Ops*. ( d ) as in a , for Rho*. ( e ) Graph of the fit constant α for the equation P (≥1 scramblase)=1−exp(−PPR/ α ) as a function of the size of the multimer being reconstituted (n-mer). Predicted values for the reconstitution of opsin monomers, dimers, tetramers and octamers are shown as blue squares (the dashed line connecting the squares is intended to guide the eye). Measured fit constants for Ops, Ops* and Rho* (taken from the data in a , c , d ) are indicated by filled circles. Full size image The fit constant α of the exponential function P (≥1 scramblase)=1−exp(−PPR/ α ) is the PPR at which 63% of the vesicles in the ensemble contain ≥1 scramblase. It also corresponds to the PPR at which each vesicle contains one reconstituted scramblase on average. For the reconstitution of Ops monomers (~42 kDa for our constructs) into 200-nm-diameter vesicles, a value for α of 0.12 mg mmol −1 can be calculated (‘Methods’) [13] ; for reconstitution of Ops multimers, α would be proportionately higher as shown in Fig. 3e (blue squares). Surprisingly, we found that the α value for the Ops data set ( Fig. 3a ) is 0.36 mg mmol −1 , which is consistent with the insertion of a mixture of preformed Ops dimers and tetramers during reconstitution ( Fig. 3e ). This result can be readily visualized by comparing the mono-exponential fit of the P (≥1 scramblase) versus PPR plot, with modelled data for the insertion of Ops monomers, dimers and tetramers ( Supplementary Fig. 3a ). The mono-exponential fits to the Ops* and Rho* data sets also yielded α values >0.12 mg mmol −1 : thus, for Ops* and Rho* we obtained α values of 0.23 and 0.43 mg mmol −1 , respectively, suggesting that these proteins—like Ops—reconstitute as small multimers ( Fig. 3e , and Supplementary Fig. 3b,c ). To understand why Ops, Ops* and Rho* reconstitute as dimers or higher order oligomers even though they are purified as monomers in DDM (ref. 43 ), we considered the possibility that the oligomeric forms are generated as detergent is withdrawn during the process of vesicle reconstitution. To test this possibility we used a previously described chemical cross-linking approach [44] ( Supplementary Fig. 4a,b ). As Ops, Ops* and Rho* are heterogeneously N -glycosylated when expressed in COS-7 cells and therefore difficult to monitor in cross-linking experiments by SDS–polyacrylamide gel electrophoresis, we used bovine rod outer segment disc rhodopsin (Rho ros ) to test our hypothesis ( Supplementary Fig. 4c ). No cross-linked adducts were detected in disc samples that were exposed to a high amount of DDM, consistent with Rho ros being monomeric when fully solubilized ( Supplementary Fig. 4c , compare lanes 3 and 4). However, dimers and higher order multimers of Rho ros were formed when the cross-linker was applied to discs that had been treated with a low amount of DDM ( Supplementary Fig. 4c , compare lane 4 with lanes 5 and 11). Thus, Rho ros multimers occur natively in disc membranes and can be detected by chemical cross-linking. To mimic vesicle reconstitution, we treated fully solubilized Rho ros with Bio-Beads to remove DDM ( Supplementary Fig. 4d ). As expected, at an early stage of detergent removal, Rho ros could not be cross-linked consistent with it being monomeric, but as detergent removal progressed cross-linking of Rho ros was evident, indicating the formation of dimers ( Supplementary Fig. 4e ). These results suggest that Ops, Ops* and Rho* are DDM-solubilized monomers at the start of the reconstitution process, and that they dimerize and oligomerize as detergent is withdrawn such that they enter vesicles as higher order structures. RhoWT scrambles phospholipids To test the scramblase activity of light-sensitive RhoWT ( Fig. 1 ) we modified our assay protocol ( Fig. 4a , ‘Dark Assay’) such that samples were maintained under dim red light during purification, reconstitution and dithionite addition, as well as during a final buffer exchange step necessary to remove unreacted dithionite. The samples were subsequently handled under room light and taken for fluorescence measurement. Mock-treated samples (no dithionite added) were analyzed in parallel. In samples of protein-free vesicles, dithionite reduced 39.7±1.5% ( n =10) of the NBD-phospholipid fluorescence ( Fig. 4b , traces labelled L; the figure shows an example from an experiment where the extent of reduction was ~35–40%), whereas ~58.5 and ~56% of NBD-PE and NBD-PC, respectively, were reduced in RhoWT-vesicles reconstituted at a PPR of ~0.5 mg mmol −1 ( Fig. 4b , red (NBD-PE) and blue (NBD-PC) end-point traces labelled P). 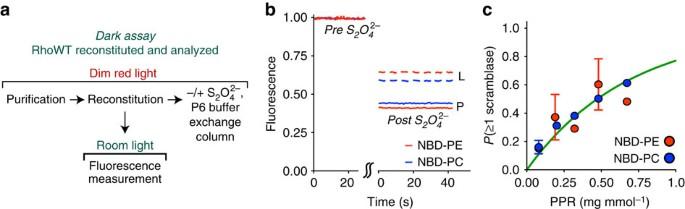Figure 4: RhoWT scrambles phospholipids. (a) ‘Dark’ assay for phospholipid scramblase activity. RhoWT is purified and reconstituted under dim red light. Also under dim red light, the reconstituted proteoliposomes are treated with dithionite, and unreacted dithionite is removed by buffer exchange on a Bio-Gel P6 column, prior to fluorescence measurements. (b) Fluorescence traces before and after dithionite treatment, detailed above, for liposomes (L; dashed lines) and RhoWT proteoliposomes at a PPR of ~1.2 mg mmol−1(P; solid lines), with either NBD-PE (red lines) or NBD-PC (blue lines) probes. (c) RhoWT was reconstituted at different PPRs and assayed under dim red light using NBD-PE or NBD-PC as indicated. The green line through the points is a mono-exponential fit of the combined data generated from both reporters. The data are graphed as mean±s.e.m. (n=2 or 4 replicates). Figure 4: RhoWT scrambles phospholipids. ( a ) ‘Dark’ assay for phospholipid scramblase activity. RhoWT is purified and reconstituted under dim red light. Also under dim red light, the reconstituted proteoliposomes are treated with dithionite, and unreacted dithionite is removed by buffer exchange on a Bio-Gel P6 column, prior to fluorescence measurements. ( b ) Fluorescence traces before and after dithionite treatment, detailed above, for liposomes (L; dashed lines) and RhoWT proteoliposomes at a PPR of ~1.2 mg mmol −1 (P; solid lines), with either NBD-PE (red lines) or NBD-PC (blue lines) probes. ( c ) RhoWT was reconstituted at different PPRs and assayed under dim red light using NBD-PE or NBD-PC as indicated. The green line through the points is a mono-exponential fit of the combined data generated from both reporters. The data are graphed as mean±s.e.m. ( n =2 or 4 replicates). Full size image The extent of dithionite-mediated reduction in protein-free vesicles using the ‘Dark Assay’ ( Fig. 4a ) was consistently lower than that obtained with a matched sample using the standard assay; likewise, the extent of reduction with RhoWT-containing vesicles was ~7–10% lower than that observed with Ops, Ops* and Rho* vesicles prepared at an equivalent PPR (see Fig. 3a,c,d ). To understand the basis for this offset we further modified our assay protocol ( Supplementary Fig. 5 ): RhoWT was purified and reconstituted under dim red light as before, but the vesicles were exposed to yellow light for at least 1.5 h before being taken for the dithionite reduction assay. By this procedure we reconstituted RhoWT but assayed bleached forms of rhodopsin comprising inactive and active conformations with respect to G protein activation, and also avoided the buffer exchange step designed to remove dithionite in the ‘Dark Assay’ protocol ( Fig. 4a ). Under these conditions, the offset in the extent of reduction was no longer observed ( Supplementary Fig. 5 ). This result suggests that the observed offset may be a consequence of the buffer exchange step in the ‘Dark Assay’ protocol. We used data obtained from the ‘Dark Assay’ protocol to generate a plot of P (≥1 scramblase) versus PPR as described above. A mono-exponential fit of the data yielded a fit constant α =0.78 mg mmol −1 , consistent with reconstitution of RhoWT into vesicles as a higher order multimer ( Supplementary Fig. 3d,e ). As discussed above, multimerization likely occurs in the final stages of detergent withdrawal during reconstitution ( Supplementary Fig. 4 ). To determine whether rhodopsin’s phospholipid scrambling activity could be generalized to other GPCR, we reconstituted carazolol-bound β 2 -adrenergic receptor and ZM 241385-bound adenosine A 2A receptor [45] , [46] . As shown in Supplementary Fig. 6 , both proteins displayed phospholipid scrambling activity. Our results place strong constraints on the mechanism by which rhodopsin transports phospholipids. We show that scrambling does not require a particular conformational state of the protein, that is, scrambling is a constitutive activity of rhodopsin, nor does it require the protein to undergo large conformational changes such as those that occur when rhodopsin is converted to metarhodopsin II. Each rhodopsin molecule facilitates the bidirectional translocation of >10 4 phospholipids per second in our reconstituted system. Such a high rate is unlikely to require large-scale conformational changes in membrane protein structure that occur typically with a frequency of ~10 3 s −1 (ref. 47 ), and is more likely to involve a transverse diffusion mechanism, where the lipid headgroup moves through a presumably solvated environment as the lipid re-orients across the bilayer. We previously proposed that conserved water molecules in the interior of opsin’s heptahelical bundle could provide a route to translocate phospholipids [13] : the headgroup of the lipid would interact with the waters while its acyl chains penetrated between TM helices to remain in the membrane interior. Our present results suggest that this mechanism is unlikely: while conserved waters are also found in RhoWT and Rho*, the Schiff base-linked retinal in these structures lies across the potential water-containing transport pathway [36] , [48] , [49] and would likely prevent the continuous transit of lipid headgroups. In addition, and independently of bound retinal, a central pathway is plugged at the luminal side of the bundle by the E2 loop ( Fig. 5a , olive loop) that is held in place by an N-terminal cap formed from residues 1–36 ( Fig. 5a , red loop). The cap and plug effectively prevent bulk solvent from accessing the retinal binding pocket and hydrolyzing the retinal Schiff base linkage [30] . The presence of the N2C/D282C disulphide bond permanently fixes the cap and plug in place, thus further restricting potential movement of phospholipids through the bundle interior in Ops, Ops*, Rho* and RhoWT. 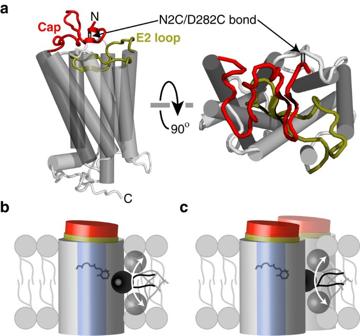Figure 5: A model for phospholipid scrambling by rhodopsin. (a) Representation of rhodopsin (based on PDB 1U19). Left, helices 1–4 are at the front of the structure. Helix 8, at the bottom of the structure, projects towards the viewer. The N-terminal residues 1–36 (red) and E2 loop (olive) form a cap and plug on the luminal side of the protein that prevents bulk solvent from entering and exchanging with conserved structural waters within the helical bundle. The engineered N2C/D282C disulphide bond is indicated. Right, a view of the same structure rotated 90° towards the reader to illustrate how the N terminus (red) and E2 loop (olive) form a cap and plug on top of the helical bundle. (b) A model for phospholipid scrambling mediated by a rhodopsin monomer. Specific features of the protein lower the energy barrier for scrambling by either thinning the bilayer, facilitating water penetration, or providing a continuous surface for lipid headgroups. The translocation route for phospholipids may involve specific features of the protein surface as depicted, or rely on packing defects generated by the protein in its immediate vicinity. Our results rule out a model in which phospholipid headgroups are translocated solely through the core of the heptahelical bundle that contains bulk water (blue cylinder): the luminal side of the bundle interior is blocked by the presence of an N-terminal cap and E2 loop (coloured as ina) in all constructs tested, and passage along the core would be additionally blocked by retinal in RhoWT and Rho* (black sticks). (c) A model for phospholipid scrambling mediated by a rhodopsin dimer. As inbexcept that the necessary surface features are provided by helices from both protomers such that scrambling requires the dimer interface. Figure 5: A model for phospholipid scrambling by rhodopsin. ( a ) Representation of rhodopsin (based on PDB 1U19). Left, helices 1–4 are at the front of the structure. Helix 8, at the bottom of the structure, projects towards the viewer. The N-terminal residues 1–36 (red) and E2 loop (olive) form a cap and plug on the luminal side of the protein that prevents bulk solvent from entering and exchanging with conserved structural waters within the helical bundle. The engineered N2C/D282C disulphide bond is indicated. Right, a view of the same structure rotated 90° towards the reader to illustrate how the N terminus (red) and E2 loop (olive) form a cap and plug on top of the helical bundle. ( b ) A model for phospholipid scrambling mediated by a rhodopsin monomer. Specific features of the protein lower the energy barrier for scrambling by either thinning the bilayer, facilitating water penetration, or providing a continuous surface for lipid headgroups. The translocation route for phospholipids may involve specific features of the protein surface as depicted, or rely on packing defects generated by the protein in its immediate vicinity. Our results rule out a model in which phospholipid headgroups are translocated solely through the core of the heptahelical bundle that contains bulk water (blue cylinder): the luminal side of the bundle interior is blocked by the presence of an N-terminal cap and E2 loop (coloured as in a ) in all constructs tested, and passage along the core would be additionally blocked by retinal in RhoWT and Rho* (black sticks). ( c ) A model for phospholipid scrambling mediated by a rhodopsin dimer. As in b except that the necessary surface features are provided by helices from both protomers such that scrambling requires the dimer interface. Full size image The constraints described above suggest that the pathway for transbilayer transit of phospholipids occurs at or near the surface of rhodopsin’s TM helical bundle ( Fig. 5b ). While there is no obviously hydrophilic transverse path on the surface of rhodopsin that could interact with phospholipid headgroups, molecular dynamics simulations support the proposal that rhodopsin lowers the energy barrier for lipid translocation and provides a transport route near its surface [50] . A similar proposal was recently made with respect to the phospholipid transport pathway of the P 4 -ATPase Atp8a2 (ref. 51 ). Here a seam along one side of the protein’s TM region was suggested to provide a water-lined route for the transiting phospholipid headgroup. An alternative mechanism invokes packing defects in the vicinity of the protein. Kol et al. [52] suggested that scramblases might operate by creating ‘flip-flop’ sites as a result of the dynamic interaction of specific TM helices with the membrane. These sites can be envisaged as packing defects in the membrane bilayer induced by TM helix movement, localized thinning of the membrane and even transient penetration of water into the bilayer from both sides. As a result of the discontinuity in lipid–lipid interactions at the lipid–protein interface, a lipid may ‘slip’ into the hydrophobic interior of the membrane with its headgroup in a solvated state, and ‘pop’ out on the other side. It seems likely that such a ‘slip-pop’ mechanism would depend on the ability of the helices, via features including their primary sequence and spatial arrangement, to engage dynamically with the membrane [53] . It remains to be seen whether such a mechanism applies to rhodopsin. All the constructs that we tested appear to integrate into vesicles as preformed multimers ranging in size from 2–6 monomers depending on the construct ( Fig. 3e ). As our DDM-solubilized constructs are likely to be monomeric [43] , [44] , [54] , it seems likely that the monomers associate in the final stages of detergent withdrawal during reconstitution such that they reconstitute as small multimers. This is consistent with our dithiobis[succinimidyl propionate] (DSP) cross-linking data ( Supplementary Fig. 4 ): at molar ratios of DDM to rhodopsin ≥300:1, or ≥2.4 micelles per rhodopsin [44] , opsin monomers are too far apart to be cross-linked. As detergent is withdrawn, the number of rhodopsins per micelle increases, and the monomers move within the 1.2 nm radius necessary for DSP cross-linking, yielding dimeric adducts that are also seen natively in disc membranes ( Supplementary Fig. 4c,e ) [44] . Similar to this conclusion, a number of previous studies showed that other GPCRs that are monomeric in detergent micelles, multimerize during reconstitution [55] , [56] , [57] . While we cannot distinguish whether the monomeric components of the reconstituted multimer are individually able to translocate phospholipids, our results raise the possibility that the phospholipid translocation pathway may require a dimer interface ( Fig. 5c ). Although the nature of rhodopsin dimerization and multimerization is imperfectly understood, a number of experimental and theoretical studies describe potential dimerization interfaces [58] , [59] , [60] . The deployment of techniques to disrupt these interfaces [61] and test the scramblase activity of monomeric rhodopsin is an objective for future work. The ability to translocate phospholipids appears to be a general property of rhodopsin-like Class A GPCRs. We have previously shown that the β 1 -adrenergic receptor has scramblase activity [13] , and we now demonstrate that the β 2 -adrenergic and adenosine A 2A receptors also scramble phospholipids ( Supplementary Fig. 6 ). GPCRs are mainly located in the plasma membrane where their scramblase activity is likely to be suppressed. The plasma membrane, like the membranes of late secretory organelles, has a characteristic bulk lipid composition marked by a high level of sphingolipids and cholesterol. It is also a thick bilayer with few packing defects, consistent with its barrier function [62] . These features may contribute to silencing the proposed constitutive scramblase activity of GPCRs. In contrast, the thin, cholesterol-poor membranes of early secretory organelles, including the ER, may provide a permissive environment for GPCR scramblase activity. In this regard, it is intriguing that the KDEL receptor, a resident of the ER and early secretory pathway, is predicted to have a GPCR-like protein fold [63] . This receptor, and perhaps GPCRs en route to the plasma membrane, may provide the phospholipid scramblase activity that is necessary for the biogenic function of the ER (refs 1 , 2 , 3 , 10 ), as well as function in membrane re-modelling in the early secretory pathway. Future studies will determine whether this is the case. Materials Egg PC, egg phosphatidic acid, NBD-PE, and NBD-PC were from Avanti Polar Lipids (Alabaster, AL, USA); Bio-Beads SM2 adsorbents (Bio-beads) and Bio-Spin chromatography columns were from Bio-Rad (Hercules, CA, USA); DSP and Micro-Spin columns with screw caps were from Thermo Scientific (Rockford, IL, USA); 100 × protease inhibitor cocktail was from EMD Millipore (Billerica, MA, USA); DDM was from Affymetrix (Maumee, OH, USA); TX from Roche Applied Science (Indianapolis, IN, USA); 9- cis -retinal, carazolol, ZM 241385, cholesteryl hemisuccinate, anti-FLAG M2 agarose, 3xFLAG peptide and anti-FLAG antibodies for immunoblotting were from Sigma (St Louis, MO, USA); PfuUltra II DNA polymerase was from Agilent (Santa Clara, CA, USA); QiaFilter Plasmid Maxi kit was from Qiagen (Valencia, CA, USA); DMEM, 100 × penicillin/streptomycin and 2-NBDG were from Invitrogen (Grand Island, NY, USA); heat-inactivated foetal bovine serum was from Atlanta Biologicals (Lawrenceville, GA, USA); 25-kDa MWCO dialysis tubing from Spectrum Laboratories (Rancho Dominguez, CA, USA); anti-mouse immunoglobulin-G horseradish peroxidase conjugate from Promega (Madison, WI, USA); 11- cis -retinal, rod cell outer segment discs and anti-1D4 were generously provided by Tom Sakmar (The Rockefeller University). Construction of mammalian expression vectors All modifications to the synthetic bovine rhodopsin gene [64] were accomplished by two-step overlap extension PCR and cloned into the NotI/EcoRI sites of the pMT3 vector [65] . The N2C and D282C mutations [37] were introduced using the gene specific forward primer 5′-gaatt gaattc caccatg tgc ggtaccgaaggccca-3′ (EcoRI cloning site underlined, mutation in bold), and the mutagenic primer 5′-cacccatcagggctct tgc tttgggcccatcttc-3′ centred at D282 (mutation in bold). The mutagenic primer for the M257Y mutation was 5′-gcgtatggttatcatc tac gtcatcgctttcctaatcgt-3′ (mutation in bold). The 3xFLAG tag sequence was cloned from the pSC211 plasmid [66] using the forward primer 5′- gcgcctgcc gactacaaggaccatgacggtgattac-3′ and reverse primer 5′-gtat gcggccgc tcacttgtcatcgtcatccttg-3′ (rhodopsin gene overlap in bold, NotI cloning site underlined) and appended to the 3′ end of the rhodopsin gene. The sequence of each of the expression vectors was verified at the Cornell University Life Sciences Core Laboratories Center. Cell culture and transfection COS-7 cells, an African green monkey kidney fibroblast-like cell line, were cultured at 37 °C in a humidified 5% CO 2 atmosphere in DMEM supplemented with 10% (v/v) heat-inactivated foetal bovine serum and 1 × penicillin/streptomycin (DMEM/FBS/PS). The cells were passaged every 3–4 days. Exponentially growing cells were harvested by trypsinization and washed once with cytomix buffer (120 mM KCl, 0.15 mM CaCl 2 , 10 mM K 2 HPO 4 /KH 2 PO 4 pH 7.6, 25 mM HEPES pH 7.6, 2 mM EGTA pH 7.6, 5 mM MgCl 2 ). The cells were subsequently resuspended at a density of 1 × 10 7 cells per ml in cytomix buffer supplemented with 2 mM ATP and 5 mM glutathione. For transfection, 20 μg of plasmid DNA and 400 μl of cell suspension were added to an ice-cold cuvette, mixed well and exposed to a single pulse of 300 V with a capacitance of 950 μF using a Bio-Rad gene pulser system. Immediately after electroporation, 1 ml of warm (37 °C) DMEM/FBS/PS was added and the sample was transferred to a 100-mm culture plate. The cells were incubated at 37 °C in a 5% CO 2 atmosphere for 48 h prior to harvesting. Immunopurification of opsins and rhodopsins Transfected COS-7 cells were harvested by washing twice in PBS and then scraping using a rubber policeman. The cells were pelleted and either used immediately or stored at −20 °C. For purification, the cell pellets were lysed in 10 mM HEPES pH 7.4, 100 mM NaCl, 19.6 mM DDM and 1 × protease inhibitor cocktail using 0.4 ml per 100-mm plate of cells, and incubated, with mixing, for 45 min at 4 °C. The resulting lysates were clarified by centrifugation at 150,000 × g for 15 min at 4 °C. To each supernatant fraction, anti-FLAG M2 agarose slurry was added (8 μl per transfected plate), and the sample was gently mixed for 2 h at 4 °C. The agarose beads were transferred to a Micro-Spin column and washed three times in 0.5 ml of buffer W (50 mM HEPES pH 7.4, 100 mM NaCl and 1.96 mM DDM). Immunopurified protein was eluted twice with 10 μl per transfected plate of Buffer W supplemented with 0.15 mg ml −1 3xFLAG peptide for 1 h at 4 °C with gentle mixing. For retinal regeneration, transfected cells were harvested and incubated overnight at 4 °C in PBS supplemented with either 5 μM 11- cis or 9- cis -retinal. Cells were pelleted and stored at −20 °C until use. All steps including and following the addition of retinal to cells were performed under dim red light. The average yield for RhoWT and RhoM257Y was ~4 μg per 10 7 cells. Rho* was generated from purified RhoM257Y after exposure to yellow light (>515 nm) for 60 s (ref. 32 ). Liposome preparation Unilamellar liposomes were prepared by a modified version of a previously reported method [13] . Briefly, chloroform stocks of egg PC (46.7 μmol), and egg phosphatidic acid (5.7 μmol) were dispensed into a round bottom flask, mixed and dried by rotary evaporation, followed by incubation for 2 h under vacuum. The lipid film was rehydrated in 10 ml of buffer A (50 mM HEPES pH 7.4, 100 mM NaCl), mixed and subjected to five freeze-thaw cycles. The suspension was extruded in a LIPEX extruder (Northern Lipids, Inc., Burnaby, BC, Canada) by 10 passes through 400-nm track-etch polycarbonate membranes followed by 4 passes through 200-nm track-etch polycarbonate membranes. The resulting liposomes (3.68±0.02 mM phospholipid, n =4, quantified as previously described [67] ) were kept at 4 °C and used within 2 weeks. For phospholipid quantification, 300 μl of perchloric acid was added to 50 μl of sample, mixed and heated at 155 °C for 60 min. After the sample was cooled to room temperature, 1 ml of water was added followed by 400 μl each of 12 g l −1 ammonium molybdate and 50 g l −1 sodium ascorbate. The sample was vortexed and heated for 10 min at 90 °C. The absorbance at 797 nm of each sample was recorded after being cooled to room temperature. Standards containing sodium phosphate were run in parallel. Proteoliposome reconstitution The reconstitution protocol was adapted from the study by Menon et al. [13] Unilamellar liposomes (800 μl) were destabilized in an 840-μl reaction containing 8.09 mM DDM in a 2-ml Eppendorf tube. After incubation for 3 h at room temperature with gentle mixing, the appropriate NBD-phospholipid probe (0.3 mole% of total phospholipid), DDM-solubilized protein and Buffer A were added such that the final 1-ml reaction contained 7 mM DDM and 2.94 mM phospholipid. The sample was mixed for an additional hour at room temperature. To form sealed vesicles, the detergent was removed by sequential addition of 80 mg Bio-beads and end-over-end mixing for 1 h at room temperature (RT), followed by the addition of 160 mg of beads for an additional 2 h at RT. The sample was then transferred to a glass screw-cap tube containing 160 mg of fresh Bio-beads and mixed overnight at 4 °C. The resulting proteoliposomes had undetectable levels of DDM quantified according to the study by Urbani and Warne [68] ; this indicates a DDM-to-phospholipid ratio of <1:100 that has been shown to have no detectable impact on bilayer organization [69] . Briefly, DDM was quantified by measuring the absorbance at 490 nm of a cooled reaction containing 50 μl of sample to which 250 μl 5% phenol and 600 μl concentrated sulphuric acid was added. Standards were prepared in parallel using samples containing 0.04–0.36 g l −1 DDM. The typical protein recovery for Ops, Ops* and Rho* was 71.8±0.84% ( n =5) as determined by quantitative western blotting that compared purified with reconstituted opsins across the PPR range tested indicated. Phospholipid recovery, determined as previously described [67] , was 67.4±0.5% ( n =8). Similar analyses for RhoWT proteoliposomes revealed 37.6±2.5% ( n =6) protein recovery and 73.4±1.3% ( n =6) phospholipid recovery. The goodness-of-fit ( r 2 ) for the calibration curves used for determining the amount of purified opsins ranged from 0.941 to 0.996 (only one fit had r 2 <0.986). Protein-free liposomes were reconstituted in parallel. For ‘dark’ samples all steps were carried out under dim red light. Scramblase assay Scramblase activity was assayed as previously described [13] . Briefly, 50 μl of proteoliposomes containing a NBD-phospholipid probe was diluted in 2 ml of Buffer A in a cuvette. The fluorescence intensity (excitation 470 nm and emission 530 nm) was recorded before and for 400 s after the addition of 40 μl of 1 M sodium dithionite in unbuffered 0.5 M Tris to a constantly stirred sample. Protein-free liposomes containing the same NBD-phospholipid probe were analyzed as part of each experiment. Analysis of P (≥1 scramblase) versus PPR plots End-point fluorescence reduction data from scramblase activity assays were obtained for proteoliposomes generated over a range of PPR values. The data were transformed according to the formula P (≥1 scramblase)=( y − y o )/( y max − y o ), where y o is the percent reduction obtained with liposomes (typically 45–50%), y max is the maximum percentage reduction observed (typically ~80%) and P is the probability that a particular vesicle in the ensemble is ‘scramblase active’, that is, it possesses at least one scramblase. The dependence of P (≥1 scramblase) on PPR was analyzed as follows. Definitions: f , number of scramblases used for reconstitution v , number of vesicles m , number of scramblases per vesicle (= f / v ) PPR, mg protein per mmol phospholipid To calculate P (≥1 scramblase) as a function of the PPR, we assume that reconstitution of opsin/rhodopsin molecules into vesicles occurs independently and that the vesicles are identical and may have more than one scramblase. The probability that a scramblase will be reconstituted into a particular vesicle is therefore 1/ v . On reconstituting f scramblases into an ensemble of v vesicles, the probability P ( k ) that a particular vesicle contains k scramblases is given by the binomial formula: Because f and v are both large, it is convenient to use the Poisson approximation: where m = f / v is the average number of scramblases per vesicle. The probability of a particular vesicle having no scramblases is: Therefore the probability that a vesicle has one or more scramblases, that is, active in the scramblase assay, is: The average number of scramblases per vesicle, m , is proportional to PPR and can be written as m =PPR/ α , where α is a constant with units of mg mmol −1 . Thus, The mono-exponential fit constant for a graph of P (≥1) versus PPR is α mg mmol −1 ; at this PPR value, m =1 and ~63% of the vesicles in the population possess ≥1 scramblase. If we assume that reconstitution of an opsin monomer (molecular weight 41.7 kDa) into a 200-nm-diameter vesicle confers scramblase activity to that vesicle, then α =0.122 mg mmol −1 (note: 1 mmol of phospholipids yields ~1.75 × 10 15 200 nm-diameter vesicles [70] ; 1 mg of opsin corresponds to 1.44 × 10 16 molecules; m = f / v =1 corresponds to 1.75 × 10 15 opsin molecules per mmol phospholipid or 0.12 mg mmol −1 ). Dark assay for scrambling All steps were performed under dim red light. Three-hundred microlitres of proteoliposomes and protein-free liposomes containing an NBD lipid probe were treated with 5 μl of 1 M sodium dithionite in unbuffered 0.5 M Tris and incubated for 400 s with end-over-end mixing. Two-hundred microlitres of sample was then buffer-exchanged over a Bio-Gel P6 column pre-equilibrated in Buffer A. Samples were also treated in parallel with 5 μl of 0.5 M unbuffered Tris. The fluorescence intensity (excitation 470 nm and emission 530 nm) was recorded for 50 μl of sample diluted into 2 ml of Buffer A in a constantly stirred cuvette. The fluorescence intensities recorded for reduced and mock-treated samples were normalized by quantification of recovered phospholipids as previously described [67] . Fluorescence reduction data were transformed as described in the preceding section. Protection of 2-NBDG trapped within vesicles Proteoliposomes containing trapped 2-NBDG were reconstituted as above except that 12.6 μM of 2-NBDG was added at the vesicle destabilization step. NBD-phospholipids were omitted, but ABD-PC was included as indicated. ABD-PC was generated from NBD-PC as follows: 33 nmoles of NBD-PC was reacted with a 1,000-fold molar excess of dithionite in 1:0.5:0.4 MeOH:CHCl 3 :H 2 O and incubated with end-over-end mixing for 7 min. The reaction was vortexed vigorously and centrifuged following addition of 0.5 ml each water and CHCl 3 , and the lower layer was extracted and washed twice with mock upper phase. The resultant non-fluorescent ABD phospholipid was dried under a stream of N 2 and 12.6 nmoles were added to reconstitutions following quantification of lipid recovery [67] . After Bio-bead treatment, 50 μl of vesicles was diluted in 2 ml of Buffer A in a cuvette. The fluorescence intensity of 2-NBDG was measured before and for 400 s after dithionite treatment as described previously for scramblase assays. To ensure complete chemical reduction of 2-NBDG, 10 μl of 10% (w/v) Triton X-100 was added to disrupt vesicles. In parallel, 500 μl of vesicles were added to a 2-ml Eppendorf tube to which either 10 μl of 1 M sodium dithionite in 0.5 M unbuffered Tris or 10 μl of 0.5 M unbuffered Tris. After incubation for 400 s with end-over-end mixing, the vesicles were dialyzed against three changes of 1 l Buffer A for 1 h at RT using 25-kDa MWCO membranes. The resulting pre-treated and dialyzed vesicles were assayed as for the vesicles taken directly from the Bio-beads. The fluorescence intensities of dialyzed vesicles were normalized to untreated vesicles by phosphate quantification [67] . How to cite this article : Goren, M. A. et al. Constitutive phospholipid scramblase activity of a G protein-coupled receptor. Nat. Commun. 5:5115 doi: 10.1038/ncomms6115 (2014).